dDsk2 regulates H2Bub1 and RNA polymerase II pausing at dHP1c complex target genes dDsk2 is a conserved extraproteasomal ubiquitin receptor that targets ubiquitylated proteins for degradation. Here we report that dDsk2 plays a nonproteolytic function in transcription regulation. dDsk2 interacts with the dHP1c complex, localizes at promoters of developmental genes and is required for transcription. Through the ubiquitin-binding domain, dDsk2 interacts with H2Bub1, a modification that occurs at dHP1c complex-binding sites. H2Bub1 is not required for binding of the complex; however, dDsk2 depletion strongly reduces H2Bub1. Co-depletion of the H2Bub1 deubiquitylase dUbp8/Nonstop suppresses this reduction and rescues expression of target genes. RNA polymerase II is strongly paused at promoters of dHP1c complex target genes and dDsk2 depletion disrupts pausing. Altogether, these results suggest that dDsk2 prevents dUbp8/Nonstop-dependent H2Bub1 deubiquitylation at promoters of dHP1c complex target genes and regulates RNA polymerase II pausing. These results expand the catalogue of nonproteolytic functions of ubiquitin receptors to the epigenetic regulation of chromatin modifications. Ubiquitin receptors bind ubiquitylated substrates and play a central role in protein degradation (reviewed in refs 1 , 2 , 3 ), an essential process that regulates multiple cellular functions. They stably associate with the proteasome as intrinsic subunits (Rpn10 and Rpn13), or only transiently as extraproteasomal receptors that selectively target ubiquitylated proteins to the proteasome. Ubiquitin receptors also participate in autophagy and endolysosomal protein degradation. In addition, although generally poorly understood, ubiquitin receptors also play nonproteolytic functions (reviewed in refs 2 , 4 , 5 ). In particular, it was reported that Rad23 is required for optimal nucleotide excision repair (NER) in yeast and that this requirement involves nonproteolytic functions of the 19S regulatory complex (19S-RC) of the proteasome [6] , [7] , [8] . The 19S-RC has also been shown to play nonproteolytic functions in transcription elongation [9] . Here we report a novel nonproteolytic function of the ubiquitin receptor dDsk2 in transcription regulation. dDsk2 belongs to the UBA/UbL family of extraproteasomal receptors (reviewed in refs 10 , 11 ), where the ubiquitin-associated (UBA) domain directly binds the ubiquitin moiety of ubiquitylated substrates [12] , [13] and the ubiquitin-like (UbL) domain mediates interaction with the proteasome [14] . dDsk2 is highly evolutionarily conserved from yeast to humans [10] , [15] , [16] . We show that, in addition to regulating protein stability, Drosophila dDsk2 interacts with the complex formed by the euchromatic dHP1c isoform and the transcription factors WOC and ROW [17] , [18] , [19] , localizes at promoters and is required for transcription via nonproteolytic mechanisms. Our results indicate that dHP1c complex target genes are enriched in developmental functions and show features associated with strong RNA polymerase II (RNA pol II) pausing. Originally considered a rare event, pausing of the promoter-proximal Pol IIo ser5 form phosphorylated at Ser5 in the C-Terminal Domain (CTD) is becoming increasingly recognized as a crucial step in transcription regulation (reviewed in refs 20 , 21 ), in particular of developmentally regulated and stimulus-responsive genes [22] , [23] , [24] , [25] . Specific factors such as NELF and DSIF are known to mediate pausing, and pause release requires their phosphorylation by P-TEFb. P-TEFb also regulates transition of Pol IIo ser5 into the elongating Pol IIo ser2 form, as it phosphorylates Ser2 in the CTD. Pausing of RNA pol II is accompanied by Pol IIo ser5 enrichment at promoters and results in the production of short RNAs [26] and increased reactivity with KMnO 4 , which reacts with unpaired thymines (T) and detects melted DNA at the sites of pausing [27] . We also show that, through the UBA domain, dDsk2 interacts with monoubiquitylated H2B (H2Bub1), an abundant histone modification [28] that is induced at promoters during transcription initiation by an activator-mediated recruitment of the ubiquitin E2/E3 enzymes Rad6/Bre1 and stimulates additional epigenetic modifications required for transcription, such as H3K4me3 and H3K79me3 (reviewed in refs 29 , 30 , 31 ). Later, during elongation, H2Bub1 extends along the entire coding region and facilitates progression of RNA pol II through chromatin. At promoters, H2Bub1 levels are dynamically regulated by Ubp8-dependent deubiquitylation [32] , [33] . Our results indicate that dDsk2 protects H2Bub1 against deubiquitylation by dUbp8/Nonstop and regulates the release of paused Pol IIo ser5 into productive elongation. In summary, here we report that the ubiquitin receptor dDsk2 plays a nonproteolytic function in transcription, regulating H2Bub1 deubiquitylation and RNA pol II pausing at promoters of dHP1c complex target genes. dDsk2 interacts with dHP1c and is required for transcription We and others previously reported that dHP1c interacts with the transcription factors WOC and ROW [17] , [18] . Here to identify partners of the dHP1c complex, we performed affinity purifications using stable S2 cell lines expressing ROW–TAP and TAP–WOC fused proteins. 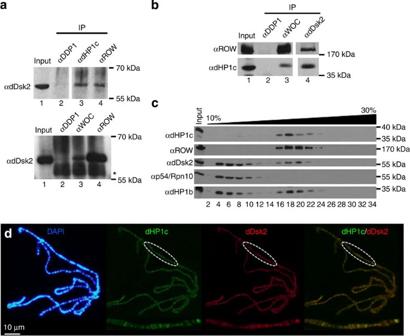Figure 1: The dHP1c complex interacts with dDsk2. (a) dDsk2 co-immunoprecipitates with components of the dHP1c complex. On the top, IPs were performed with rat polyclonal αdHP1c (lane 3), αROW (lane 4) and control αDDP1 (lane 2) antibodies. On the bottom, IPs were performed with rabbit polyclonal αWOC (lane 3), αROW (lane 4) and control αDDP1 (lane 2). IP materials were analysed by western blot analysis using rabbit polyclonal αdDsk2. Lane 1 corresponds to 2.5% of the input material. At the bottom, the asterisk (*) indicates a band corresponding to IgGs. The position of markers of known molecular weight (kDa) is indicated. (b) Components of the dHP1c complex co-immunoprecipitate with dDsk2. IPs were performed with rabbit αdDsk2 (lane 4), and control αWOC (lane 3) and αDDP1 (lane 2) antibodies, and analysed with western blot analysis using rat polyclonal αROW (top) and αdHP1c (bottom). Lane 1 corresponds to 2.5% of the input material. The position of markers of known molecular weight (kDa) is indicated. (c) Glycerol gradient (10–30%) sedimentation analysis of a total S2-cell protein extract. Fractions were collected from top to bottom and were analysed with western blot analysis using rat polyclonal αdHP1c, αdHP1b and αROW, rabbit polyclonal αdDsk2 and mouse polyclonal αp54/Rpn10. Fractions 2–34 are shown. Lane 1 corresponds to 2.5% of the input material. The position of markers of known molecular weight (kDa) is indicated. (d) dHP1c and dDsk2 strongly colocalize. Polytene chromosomes were immunostained with rat polyclonal αdHP1c (green) and rabbit polyclonal αdDsk2 (red) antibodies. Enlarged images of the indicated region are shown at the bottom. DNA was stained with DAPI (blue). Scale bar, 10 μm. Co-purified proteins identified with high confidence are listed in Table 1 . In addition to dHP1c, WOC and ROW, these experiments detected the dHP1b isoform [34] ; the boundary protein BEAF-32 (ref. 35 ); the chromosomal proteins Chromator and Z4, which are known to form a complex [36] , [37] ; the RNA-binding protein Blanks [38] ; the ubiquitin receptor protein dDsk2; and coilin, a factor that marks Cajal bodies and associates to the histone locus [39] . Co-IP experiments directly confirmed several of these interactions. In particular, a strong interaction with dDsk2 was detected, as IPs performed with αdHP1c, αWOC and αROW antibodies bring down dDsk2 ( Fig. 1a ) and, vice versa , αDsk2 antibodies co-immunoprecipitate dHP1c and ROW ( Fig. 1b ). Furthermore, glycerol gradient centrifugation shows that a significant proportion of dDsk2 co-sediments with the dHP1c complex ( Fig. 1c ). Notice that the poor performance of αWOC antibodies in western blot (WB) analyses prevented the detection of WOC in these experiments (see Methods and Supplementary Fig. 11a ). Finally, immunostaining experiments in polytene chromosomes detected a strong colocalization of dHP1c and dDsk2 ( Fig. 1d ). Table 1 Proteins co-purifying with WOC and ROW. Full size table Figure 1: The dHP1c complex interacts with dDsk2. ( a ) dDsk2 co-immunoprecipitates with components of the dHP1c complex. On the top, IPs were performed with rat polyclonal αdHP1c (lane 3), αROW (lane 4) and control αDDP1 (lane 2) antibodies. On the bottom, IPs were performed with rabbit polyclonal αWOC (lane 3), αROW (lane 4) and control αDDP1 (lane 2). IP materials were analysed by western blot analysis using rabbit polyclonal αdDsk2. Lane 1 corresponds to 2.5% of the input material. At the bottom, the asterisk (*) indicates a band corresponding to IgGs. The position of markers of known molecular weight (kDa) is indicated. ( b ) Components of the dHP1c complex co-immunoprecipitate with dDsk2. IPs were performed with rabbit αdDsk2 (lane 4), and control αWOC (lane 3) and αDDP1 (lane 2) antibodies, and analysed with western blot analysis using rat polyclonal αROW (top) and αdHP1c (bottom). Lane 1 corresponds to 2.5% of the input material. The position of markers of known molecular weight (kDa) is indicated. ( c ) Glycerol gradient (10–30%) sedimentation analysis of a total S2-cell protein extract. Fractions were collected from top to bottom and were analysed with western blot analysis using rat polyclonal αdHP1c, αdHP1b and αROW, rabbit polyclonal αdDsk2 and mouse polyclonal αp54/Rpn10. Fractions 2–34 are shown. Lane 1 corresponds to 2.5% of the input material. The position of markers of known molecular weight (kDa) is indicated. ( d ) dHP1c and dDsk2 strongly colocalize. Polytene chromosomes were immunostained with rat polyclonal αdHP1c (green) and rabbit polyclonal αdDsk2 (red) antibodies. Enlarged images of the indicated region are shown at the bottom. DNA was stained with DAPI (blue). Scale bar, 10 μm. Full size image The dHP1c complex was shown to localize at active chromatin domains, suggesting a role in gene expression regulation [17] , [18] . However, its actual genomic distribution and the extent of overlapping of its components were not known. To address these questions, we performed chromatin immunoprecipitation-sequencing (ChIP-seq) experiments to determine the genomic binding profiles of dHP1c, WOC, ROW and dDsk2. As shown in Fig. 2a , the four factors predominantly localize at promoters with ∼ 60% of peaks lying within ±1 kb to a transcription start site (TSS). The distributions of dHP1c, WOC and dDsk2 are centred at TSS and largely overlap, whereas ROW shows a bimodal distribution with a major peak slightly displaced downstream from the TSS and a second peak localizing ∼ 0.5 kb upstream ( Fig. 2b ). The four factors strongly colocalize ( Fig. 2c ), with more than 1,500 common target genes identified. Common genes account for a high proportion ( ∼ 70%) of dHP1c targets but, on the other hand, they constitute a much lower proportion of WOC ( ∼ 30%), ROW ( ∼ 25%) and dDsk2 ( ∼ 35%) targets. These differences appear to largely arise from the different performance of the antibodies used in ChIP experiments since dHP1c is detected at WOC/ROW/dDsk2 target genes regardless of whether they are statistically identified as dHP1c targets or not. Indeed, dHP1c abundance at these genes is higher than at non-WOC/ROW/dDsk2 target genes ( Supplementary Fig. 1a ) and its distribution is similar to that observed in target genes ( Supplementary Fig. 1b ). Furthermore, ChIP-chip data generated by the modENCODE project identify a higher number of dHP1c target genes ( Supplementary Fig. 1c ), a majority of which is also detected as WOC/ROW/dDsk2 targets in our experiments ( Supplementary Fig. 1d ). 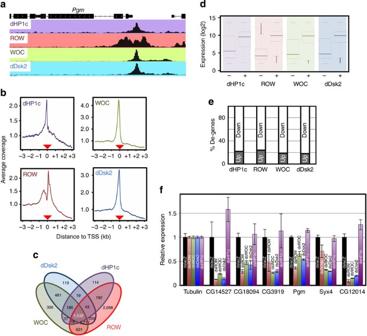Figure 2: The dHP1c complex localizes at TSS and is required for transcription. (a) ChIP-seq coverage profiles of dHP1c, ROW, WOC and dDsk2 across a representative region. Genomic organization of the region is indicated. Antibodies used were rabbit polyclonal αdHP1c, αROW, αWOC and αdDsk2. (b) The distribution around TSS is presented for dHP1c, ROW, WOC and dDsk2. For each gene, the coverage profile was normalized dividing by the average coverage in that gene. The position of the TSS is indicated. (c) Venn diagram showing the intersection between dHP1c, ROW, WOC and dDsk2 target genes. (d) Box plot showing the expression in S2 cells of dHP1c, ROW, WOC and dDsk2 target (+) and non-target (−) genes. (e) The percentage of dHP1c, ROW, WOC and dDsk2 target genes that are found to be differentially down- and upregulated on depletion of ROW in S2 cells is presented. (f) mRNA levels of six dHP1c complex target genes are determined by RT–qPCR in S2 cells on depletion of dHP1c (purple), ROW (red), WOC (green) and dDsk2 (blue). mRNA levels were determined in relation to cells treated with dsRNA against LacZ (black). Results were normalized with respect to Tubulin levels. (Number of experimental replicates,N=4). Error bars correspond to s.d. Figure 2: The dHP1c complex localizes at TSS and is required for transcription. ( a ) ChIP-seq coverage profiles of dHP1c, ROW, WOC and dDsk2 across a representative region. Genomic organization of the region is indicated. Antibodies used were rabbit polyclonal αdHP1c, αROW, αWOC and αdDsk2. ( b ) The distribution around TSS is presented for dHP1c, ROW, WOC and dDsk2. For each gene, the coverage profile was normalized dividing by the average coverage in that gene. The position of the TSS is indicated. ( c ) Venn diagram showing the intersection between dHP1c, ROW, WOC and dDsk2 target genes. ( d ) Box plot showing the expression in S2 cells of dHP1c, ROW, WOC and dDsk2 target (+) and non-target (−) genes. ( e ) The percentage of dHP1c, ROW, WOC and dDsk2 target genes that are found to be differentially down- and upregulated on depletion of ROW in S2 cells is presented. ( f ) mRNA levels of six dHP1c complex target genes are determined by RT–qPCR in S2 cells on depletion of dHP1c (purple), ROW (red), WOC (green) and dDsk2 (blue). mRNA levels were determined in relation to cells treated with dsRNA against LacZ (black). Results were normalized with respect to Tubulin levels. (Number of experimental replicates, N =4). Error bars correspond to s.d. Full size image Expression profiling analyses indicate that the dHP1c complex is required for transcription since target genes are actively transcribed ( Fig. 2d ) and, on RNA interference (RNAi)-mediated depletion of ROW, ∼ 80% of the target genes changing expression are found to be downregulated ( Fig. 2e ). Reverse transcription–quantitative PCR (RT–qPCR) experiments confirmed these results since several selected target genes were found to be significantly downregulated on ROW depletion (3.9 × 10 −8 < P <0.017, Student’s t -test; Fig. 2f ). WOC and dDsk2 depletion led to a similar effect on expression but, in contrast, no such downregulation was observed on dHP1c depletion ( Fig. 2f ). In this regard, we observed that dHP1b co-purifies with WOC and ROW ( Table 1 ), co-sediments ( Fig. 1c ) and co-immunoprecipitates with dHP1c, ROW and dDsk2 ( Supplementary Fig. 2c ), and highly overlaps with dHP1c at promoters ( Supplementary Fig. 2a,b ), suggesting that it could compensate the loss of dHP1c. However, although co-depletion of dHP1c and dHP1b tends to affect gene expression more than single dHP1c depletion ( Supplementary Fig. 2d ), the observed effects are weaker than when WOC, ROW or dDsk2 are depleted ( Fig. 2f ). Gene ontology analyses show that dHP1c complex target genes are enriched in developmental functions ( Fig. 3a ). RNA pol II pausing is generally high at developmentally regulated genes [22] , [23] , [24] , [25] . Accordingly, dHP1c complex target genes show features of strong RNA pol II pausing ( Fig. 3b ). In comparison with non-target genes, the distribution of total RNA pol II (RPB1) is strongly biased towards the TSS. Consequently, the pausing index (PI), determined as the ratio of total RNA pol II abundance at TSS±250 bp with respect to the last 500 bp of the gene [24] , is significantly higher ( P <0.0001, Kruskal–Wallis; Fig. 3b ). Concomitantly, Pol IIo ser5 is enriched at promoters of ∼ 50% of dHP1c complex target genes ( Fig. 3c , left). In addition, target genes are enriched in NELF ( Fig. 3c , centre) and short RNAs resulting from RNA pol II pausing are detected in as many as ∼ 93% of them ( Fig. 3c , right). Furthermore, KMnO 4 reactivity is detected in ∼ 94% of target genes ( Fig. 3d , left). Most importantly, target genes are strongly hyper-reactive to KMnO 4 since ∼ 40% of them show reactivity above the third quartile, in front of the expected 25% ( P <0.0001, Benjamini–Yekutieli-adjusted Fisher exact test; Fig. 3d , right). This enrichment is similar to that observed for Pol IIo ser5 target genes and significantly higher than for NELF targets ( P <0.0001, Benjamini–Yekutieli-adjusted Fisher exact test; Fig. 3d , right). 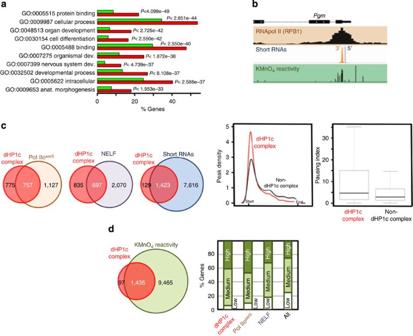Figure 3: dHP1c complex target genes are enriched in developmental functions and show strong RNA pol II pausing. (a) The percentages of dHP1c complex target (red) and non-target genes (green) are shown for the 10 most enriched functions. Statistical significance of the differences (Benjamini–Yekutieli-adjusted Fisher exact testPvalue) is indicated. (b) On the top, the coverage profiles across a representative region are presented for total RNA pol II (RPB1), short RNAs and KMnO4reactivity. Genomic organization of the region is indicated. On the bottom, the distribution of total RNA pol II (RPB1) across a standardized gene (left) and a box plot showing the RNA pol II pausing index (right) are presented for dHP1c complex target (red) and non-target (black) genes. (c) Venn diagrams showing the intersection between dHP1c complex target genes and Pol IIoser5(left), NELF-E (centre) and short RNA (right) target genes. (d) On the left, a Venn diagram showing the intersection between dHP1c complex target genes and genes showing significant KMnO4reactivity is presented. On the right, the percentage of dHP1c complex target genes showing low (min to first quartile; white), medium (first to third quartile; light green) and high (third quartile to max; dark green) KMnO4reactivity is compared with NELF-E and Pol IIoser5target genes, and all genes. Figure 3: dHP1c complex target genes are enriched in developmental functions and show strong RNA pol II pausing. ( a ) The percentages of dHP1c complex target (red) and non-target genes (green) are shown for the 10 most enriched functions. Statistical significance of the differences (Benjamini–Yekutieli-adjusted Fisher exact test P value) is indicated. ( b ) On the top, the coverage profiles across a representative region are presented for total RNA pol II (RPB1), short RNAs and KMnO 4 reactivity. Genomic organization of the region is indicated. On the bottom, the distribution of total RNA pol II (RPB1) across a standardized gene (left) and a box plot showing the RNA pol II pausing index (right) are presented for dHP1c complex target (red) and non-target (black) genes. ( c ) Venn diagrams showing the intersection between dHP1c complex target genes and Pol IIo ser5 (left), NELF-E (centre) and short RNA (right) target genes. ( d ) On the left, a Venn diagram showing the intersection between dHP1c complex target genes and genes showing significant KMnO 4 reactivity is presented. On the right, the percentage of dHP1c complex target genes showing low (min to first quartile; white), medium (first to third quartile; light green) and high (third quartile to max; dark green) KMnO 4 reactivity is compared with NELF-E and Pol IIo ser5 target genes, and all genes. Full size image dDsk2 plays a nonproteolytic function in the dHP1c complex The contribution of the proteasome to transcription regulation has been extensively documented (reviewed in refs 40 , 41 , 42 ). In particular, proteasome-mediated degradation has been shown to directly affect transcription by coupling transcription factor turnover to activation. Thus, considering its role in targeting substrates to the proteasome for degradation, we addressed the possibility that dDsk2 could mediate dHP1c complex recruitment to the proteasome and degradation. However, opposite to this hypothesis, dDsk2 depletion in S2 cells does not increase stability of the complex; however, it results in a slight decrease in total dHP1c and ROW content ( Fig. 4a ). Immunostaining experiments in wing imaginal discs confirmed these results. In these experiments, we used dsk2 RNAi flies to specifically deplete dDsk2 at the anterior/posterior (A/P) border using a ptc -GAL4 driver. Under these conditions, dDsk2 depletion is strong and slightly reduces dHP1c, WOC and ROW levels, whereas no such reduction is detected at the A/P border of control flies ( Fig. 4b ). Moreover, co-IP experiments failed to detect an interaction with p54/Rpn10, the proteasome subunit that mediates dDsk2 binding [10] , [11] , [43] , [44] ( Fig. 4c ). Similarly, glycerol gradient centrifugation showed no detectable p54/Rpn10 co-sedimenting together with the dHP1c complex ( Fig. 1c ). In addition, an interaction with the proteasome is unlikely since the UbL domain is required for both binding to the proteasome [10] , [11] and assembly into the dHP1c complex, as αHP1c and αROW antibodies co-immunoprecipitate overexpressed full-length dDsk2 ( Fig. 4d , lanes dDsk2), but not a truncated form missing the UbL domain ( Fig. 4d , lanes ΔUbL). In contrast, deleting the UBA domain has no effect ( Fig. 4d , lanes ΔUBA), indicating that it is dispensable for assembly into the dHP1c complex. 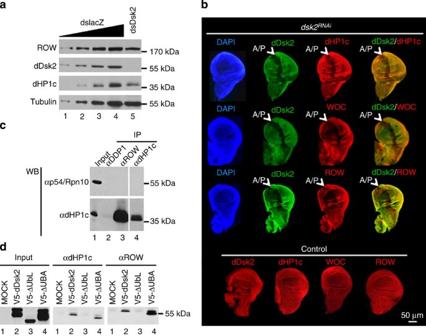Figure 4: dDsk2 does not mediate proteolytic degradation of the dHP1c complex. (a) The levels of ROW, dHP1c and dDsk2 are determined using western blot analysis in extracts prepared from control S2 cells treated with dsRNA against LacZ (lanes 1–4: increasing amounts of extract are analysed) and on depletion of dDsk2 (lane 5). Tubulin levels are also presented as loading control. Antibodies used were rabbit polyclonal αROW and αDsk2, rat polyclonal αdHP1c and mouse αTubulin. The position of markers of known molecular weight (kDa) is indicated. (b) On the top, wing imaginal discs obtained fromdsk2RNAi; ptc-GAL4 larvae were immunostained with rabbit polyclonal αdDsk2 (green) and rat polyclonal αHP1c (top), αWOC (centre) and αROW (bottom) antibodies (red). DNA was stained with 4,6-diamidino-2-phenylindole (DAPI, blue). The arrows indicate the A/P boundary where theptcpromoter is specifically active. On the bottom, wing imaginal discs obtained from control wild-type larvae were stained with rabbit polyclonal αdDsk2 and rat polyclonal αHP1c, αWOC and αROW antibodies (in red). Scale bar, 50 μm. (c) p54/Rpn10 does not co-immunoprecipitate with the dHP1c complex. IPs were performed with rabbit polyclonal αROW (lane 3), αdHP1c (lane 4) and control αDDP1 (lane 2) antibodies. IP materials were analysed by western blot using mouse polyclonal αp54/Rpn10 (top) and rat polyclonal αdHP1c (bottom). Lane 1 corresponds to 2.5% of the input material. The position of markers of known molecular weight (kDa) is indicated. (d) Nuclear extracts obtained from S2 cells expressing the indicated V5-tagged dDsk2 constructs (lanes 2–4) were subjected to immunoprecipitation with rabbit polyclonal αHP1c (centre) and αROW (right) antibodies, and analysed by western blot using mouse monoclonal αV5 antibodies. The panel on the left corresponds to 1% of the input material used in each case for the immunoprecipitation. Lane 1 corresponds to a mock extract prepared from S2 cells expressing no V5-tagged construct. The position of markers of known molecular weight (kDa) is indicated. Figure 4: dDsk2 does not mediate proteolytic degradation of the dHP1c complex. ( a ) The levels of ROW, dHP1c and dDsk2 are determined using western blot analysis in extracts prepared from control S2 cells treated with dsRNA against LacZ (lanes 1–4: increasing amounts of extract are analysed) and on depletion of dDsk2 (lane 5). Tubulin levels are also presented as loading control. Antibodies used were rabbit polyclonal αROW and αDsk2, rat polyclonal αdHP1c and mouse αTubulin. The position of markers of known molecular weight (kDa) is indicated. ( b ) On the top, wing imaginal discs obtained from dsk2 RNAi ; ptc- GAL4 larvae were immunostained with rabbit polyclonal αdDsk2 (green) and rat polyclonal αHP1c (top), αWOC (centre) and αROW (bottom) antibodies (red). DNA was stained with 4,6-diamidino-2-phenylindole (DAPI, blue). The arrows indicate the A/P boundary where the ptc promoter is specifically active. On the bottom, wing imaginal discs obtained from control wild-type larvae were stained with rabbit polyclonal αdDsk2 and rat polyclonal αHP1c, αWOC and αROW antibodies (in red). Scale bar, 50 μm. ( c ) p54/Rpn10 does not co-immunoprecipitate with the dHP1c complex. IPs were performed with rabbit polyclonal αROW (lane 3), αdHP1c (lane 4) and control αDDP1 (lane 2) antibodies. IP materials were analysed by western blot using mouse polyclonal αp54/Rpn10 (top) and rat polyclonal αdHP1c (bottom). Lane 1 corresponds to 2.5% of the input material. The position of markers of known molecular weight (kDa) is indicated. ( d ) Nuclear extracts obtained from S2 cells expressing the indicated V5-tagged dDsk2 constructs (lanes 2–4) were subjected to immunoprecipitation with rabbit polyclonal αHP1c (centre) and αROW (right) antibodies, and analysed by western blot using mouse monoclonal αV5 antibodies. The panel on the left corresponds to 1% of the input material used in each case for the immunoprecipitation. Lane 1 corresponds to a mock extract prepared from S2 cells expressing no V5-tagged construct. The position of markers of known molecular weight (kDa) is indicated. Full size image dDsk2 interacts with and regulates H2Bub1 Ubiquitin receptors usually bind ubiquitylated substrates. Thus, we addressed the possibility that, through the UBA domain, dDsk2 might recognize an ubiquitylated chromatin component. In this regard, a prominent feature of dHP1c complex-binding sites is the presence of H2Bub1 ( Fig. 5a ), suggesting that dDsk2 might interact with H2Bub1. Peptide pull-down assays support this possibility since the UBA domain of dDsk2 strongly binds a biotinylated H2B peptide encompassing the ubiquitylation site, K118 in Drosophila , only when it is ubiquitylated (H2BubK118; Fig. 5b , row UBA). Notice that full-length dDsk2 binds H2BubK118 very inefficiently ( Fig. 5b , row dDsk2), while deleting the UbL domain restores binding ( Fig. 5b , row ΔUbL). Most probably, this observation reflects the UbL–UBA self-interaction that is known to occur in vitro and blocks recognition of ubiquitylated substrates [45] . Furthermore, overexpression experiments in S2 cells showed that the UBA domain stabilizes the binding of dDsk2 to chromatin since full-length dDsk2 is detected in both the cytosolic and chromatin-bound fractions, and deleting the UBA domain reduces binding to chromatin ( Fig. 5d ). Concomitantly, overexpression of the ΔUBA–dDsk2 construct significantly downregulates expression of targets genes ( P <0.01, Student’s t -test; Fig. 5e ), which is similar to the effect of dDsk2 depletion, indicating that the truncated ΔUBA–dDsk2 form has a dominant-negative character. Notice that the ΔUBA–dDsk2 form assembles efficiently into the dHP1c complex ( Fig. 4d ). However, reducing H2Bub1 levels by Rad6/Bre1 depletion has only a weak effect on binding of dDsk2, WOC and ROW ( Fig. 5f ). Altogether, these results suggest that, although the interaction of dDsk2 with H2Bub1 is important for transcription and stabilizes binding of the complex, it is not essential for its recruitment to promoters. In this regard, the zinc-finger proteins WOC and ROW mediate binding of both dHP1c [18] and dDsk2 ( Supplementary Fig. 3a,b ), suggesting that they play a crucial role in recruitment. However, although largely independent of the interaction with H2Bub1, binding of the complex also requires dDsk2 ( Supplementary Fig. 3c,d ). 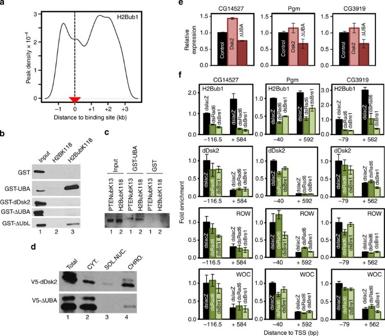Figure 5: The UBA domain of dDsk2 binds H2Bub1. (a) H2Bub1 distribution at binding sites of the dHP1c complex as determined from ChIP-chip data generated with the modENCODE project (ID 290). Binding sites of the dHP1c complex were oriented with respect to the direction of transcription of the closest gene. Peak density is presented as a function of the distance to the centre of the binding site. (b) The indicated recombinant GST-tagged dDsk2 constructs were assayed for binding to a biotinylated H2B peptide (aa104–123) carrying ubiquitylated K118 (H2BubK118; lanes 3) or not (H2BK118; lanes 2). Binding was analysed by peptide pull-down using streptavidin–sepharose beads and western blot analysis of the bound material using αGST antibodies. Lane 1 corresponds to 1% of the GST constructs used in the binding experiments. The position of markers of known molecular weight (kDa) is indicated. (c) The binding of the UBA domain of dDsk2 to H2BubK118 (lanes 2) and a PTENubK13 peptide (aa5–21) ubiquitylated at K13 was determined by GST pull-down assays with the indicated GST constructs using glutathione sepharose 4B beads. Binding was analysed with western blot analysis using mouse αubiquitin. The position of markers of known molecular weight (kDa) is indicated. (d) The indicated V5-tagged dDsk2 constructs were overexpressed in S2 cells. Extracts were fractionated into cytosolic (CYT.; lanes 2), soluble nuclear (SOL.NUC.; lanes 3) and chromatin-bound (CHRO.; lanes 4) fractions, and analysed by western blot using mouse monoclonal αV5 antibodies. Lane 1 corresponds to a total extract prepared from S2 cells expressing the indicated V5-tagged constructs. The position of markers of known molecular weight (kDa) is indicated. (e) mRNA levels of the indicated dHP1c complex target genes are determined by RT–qPCR in S2 cells on overexpression of full-length dDsk2 (light red) and the truncated ΔUBA–dDsk2 form missing de UBA domain (dark red). mRNA levels were determined in relation to control cells expressing no construct (black). Results were normalized with respect to Actin5C levels (N=3). (f) H2Bub1, dDsk2, ROW and WOC levels at the indicated positions with respect to TSS of selected target genes are determined by ChIP–qPCR in control S2 cells treated with dsRNA against LacZ (black), and on depletion of dRad6 (dark green) and dBre1 (light green). Results are presented as fold enrichment with respect to the control (dsLacZ) at the most upstream position. Antibodies used were mouse monoclonal αH2Bub1 and rabbit polyclonal αDsk2, αROW and αWOC (N=3). Error bars correspond to s.d. Figure 5: The UBA domain of dDsk2 binds H2Bub1. ( a ) H2Bub1 distribution at binding sites of the dHP1c complex as determined from ChIP-chip data generated with the modENCODE project (ID 290). Binding sites of the dHP1c complex were oriented with respect to the direction of transcription of the closest gene. Peak density is presented as a function of the distance to the centre of the binding site. ( b ) The indicated recombinant GST-tagged dDsk2 constructs were assayed for binding to a biotinylated H2B peptide (aa104–123) carrying ubiquitylated K118 (H2BubK118; lanes 3) or not (H2BK118; lanes 2). Binding was analysed by peptide pull-down using streptavidin–sepharose beads and western blot analysis of the bound material using αGST antibodies. Lane 1 corresponds to 1% of the GST constructs used in the binding experiments. The position of markers of known molecular weight (kDa) is indicated. ( c ) The binding of the UBA domain of dDsk2 to H2BubK118 (lanes 2) and a PTENubK13 peptide (aa5–21) ubiquitylated at K13 was determined by GST pull-down assays with the indicated GST constructs using glutathione sepharose 4B beads. Binding was analysed with western blot analysis using mouse αubiquitin. The position of markers of known molecular weight (kDa) is indicated. ( d ) The indicated V5-tagged dDsk2 constructs were overexpressed in S2 cells. Extracts were fractionated into cytosolic (CYT. ; lanes 2), soluble nuclear (SOL.NUC. ; lanes 3) and chromatin-bound (CHRO. ; lanes 4) fractions, and analysed by western blot using mouse monoclonal αV5 antibodies. Lane 1 corresponds to a total extract prepared from S2 cells expressing the indicated V5-tagged constructs. The position of markers of known molecular weight (kDa) is indicated. ( e ) mRNA levels of the indicated dHP1c complex target genes are determined by RT–qPCR in S2 cells on overexpression of full-length dDsk2 (light red) and the truncated ΔUBA–dDsk2 form missing de UBA domain (dark red). mRNA levels were determined in relation to control cells expressing no construct (black). Results were normalized with respect to Actin5C levels ( N =3). ( f ) H2Bub1, dDsk2, ROW and WOC levels at the indicated positions with respect to TSS of selected target genes are determined by ChIP–qPCR in control S2 cells treated with dsRNA against LacZ (black), and on depletion of dRad6 (dark green) and dBre1 (light green). Results are presented as fold enrichment with respect to the control (dsLacZ) at the most upstream position. Antibodies used were mouse monoclonal αH2Bub1 and rabbit polyclonal αDsk2, αROW and αWOC ( N =3). Error bars correspond to s.d. Full size image Ubiquitin receptors have also been shown to protect ubiquitylated conjugates against deubiquitylation [10] , [11] , suggesting that dDsk2–H2Bub1 interaction could prevent H2Bub1 deubiquitylation. Consistent with this hypothesis, dDsk2 depletion strongly reduces H2Bub1 at promoters of target genes ( P <0.01, Student’s t -test; Fig. 6a ). Similarly, overexpression of the ΔUBA–dDsk2 form also reduces H2Bub1 levels ( P <0.05. Student’s t -test; Fig. 6b ). Furthermore, depletion of the H2Bub1 deubiquitylase dUbp8/Nonstop suppresses this effect since, on dDsk2 and dUbp8/Nonstop co-depletion, H2Bub1 levels are higher than when only dDsk2 is depleted ( P <0.001, Student’s t -test) and similar to those observed in control cells ( Fig. 6c , top). These changes in H2Bub1 levels are not due to differential nucleosome occupancy, as H3 abundance is similar in control and knockdown conditions ( Fig. 6c , bottom). In addition, expression of target genes, which is strongly decreased on dDsk2 depletion, is significantly rescued when dUbp8/Nonstop is co-depleted ( P <0.001, Student’s t -test; Fig. 6d ), whereas binding of both WOC and ROW is not ( Fig. 6e ). 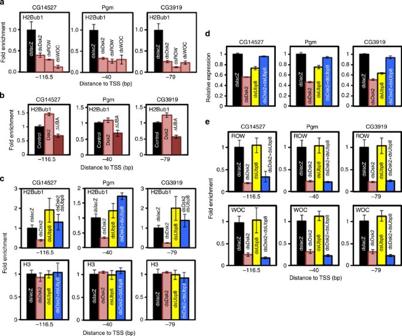Figure 6: dDsk2 regulates H2Bub1 deubiquitylation at promoters of dHP1c complex target genes. (a) H2Bub1 levels at the indicated positions with respect to TSS of selected target genes are determined by ChIP–qPCR in control S2 cells treated with dsRNA against LacZ (black) and on depletion of dDsk2, ROW and WOC (red). Results are presented as fold enrichment with respect to the control (dsLacZ). Antibodies used were mouse monoclonal αH2Bub1 (N=5). (b) As ina, but for H2Bub1 levels on overexpression of full-length dDsk2 (light red) and the truncated ΔUBA–dDsk2 form (dark red). Results are presented as fold enrichment with respect to control cells expressing no construct (black;N=3). (c) As ina, but for H2Bub1 (top) and H3 (bottom) levels on depletion of dDsk2 (red), dUbp8/Nonstop (yellow) and both (blue;N=3). (d) mRNA levels of the indicated target genes are determined by RT–qPCR in S2 cells on depletion of dDsk2 (red), dUbp8/Nonstop (yellow) and both (blue). mRNA levels were determined in relation to control cells treated with dsRNA against LacZ (black). Results were normalized with respect to Actin5C levels (N=3). (e) As ina, but for ROW (top) and WOC (bottom) levels on depletion of dDsk2 (red), dUbp8/Nonstop (yellow) and both (blue;N=3). Error bars correspond to s.d. Figure 6: dDsk2 regulates H2Bub1 deubiquitylation at promoters of dHP1c complex target genes. ( a ) H2Bub1 levels at the indicated positions with respect to TSS of selected target genes are determined by ChIP–qPCR in control S2 cells treated with dsRNA against LacZ (black) and on depletion of dDsk2, ROW and WOC (red). Results are presented as fold enrichment with respect to the control (dsLacZ). Antibodies used were mouse monoclonal αH2Bub1 ( N =5). ( b ) As in a , but for H2Bub1 levels on overexpression of full-length dDsk2 (light red) and the truncated ΔUBA–dDsk2 form (dark red). Results are presented as fold enrichment with respect to control cells expressing no construct (black; N =3). ( c ) As in a , but for H2Bub1 (top) and H3 (bottom) levels on depletion of dDsk2 (red), dUbp8/Nonstop (yellow) and both (blue; N =3). ( d ) mRNA levels of the indicated target genes are determined by RT–qPCR in S2 cells on depletion of dDsk2 (red), dUbp8/Nonstop (yellow) and both (blue). mRNA levels were determined in relation to control cells treated with dsRNA against LacZ (black). Results were normalized with respect to Actin5C levels ( N =3). ( e ) As in a , but for ROW (top) and WOC (bottom) levels on depletion of dDsk2 (red), dUbp8/Nonstop (yellow) and both (blue; N =3). Error bars correspond to s.d. Full size image dHP1c complex target genes show features associated with strong RNA pol II pausing ( Fig. 3 ). Thus, we considered the possibility that the contribution of dDsk2 to transcription reflects a role in RNA pol II pausing. To address this question, we determined the distribution of total RNA pol II (RPB3) and the promoter-proximal Pol IIo ser5 form across target genes ( Fig. 7a ). In both cases, strong accumulation is detected at TSS in control cells as well as on dUbp8/Nonstop depletion. In contrast, dDsk2 depletion reduces RPB3 and Pol IIo ser5 occupancy all across the gene. Importantly, this reduction preferentially occurs at the promoter, as relative abundance at TSS with respect to the total abundance across the gene is significantly reduced in dDsk2-depleted cells ( P <0.05, Student’s t -test; Fig. 7b ), which suggests a defect in pausing. In good agreement, dDsk2 depletion significantly reduces NELF-E occupancy at TSS ( P <0.02, Student’s t -test; Fig. 7c ). Furthermore, NELF-E depletion induces a similar decrease in RNA pol II occupancy across the gene, which is significantly stronger at TSS ( P <0.05, Student’s t -test; Supplementary Fig. 4 ). Besides, the extent of histone acetylation at the promoter remains high ( Fig. 7d ), indicating that the active chromatin configuration of the promoter is retained on dDsk2 depletion. In contrast, dDsk2 depletion induces a strong reduction of H3K4me3 at promoters ( Fig. 7d ), as expected from the reported H2Bub1–H3K4me3 crosstalk [29] , [30] , [31] . Notably, co-depletion of Ubp8/Nonstop, which rescues H2Bub1 and expression ( Fig. 6c,d ), also rescues RPB3 and Pol IIo ser5 levels at TSS ( Fig. 7a,b ). Finally, in a control gene whose expression is not affected by dDsk2 depletion ( Supplementary Fig. 5a , left), the levels of H2Bub1 ( Supplementary Fig. 5b , left), and RPB3 and Pol IIo ser5 at TSS ( Supplementary Fig. 5c ) are unchanged on dDsk2 depletion. Similarly, overexpression of the ΔUBA–dDsk2 construct does not affect expression ( Supplementary Fig. 5a , right) or H2Bub1 levels ( Supplementary Fig. 5b , right). 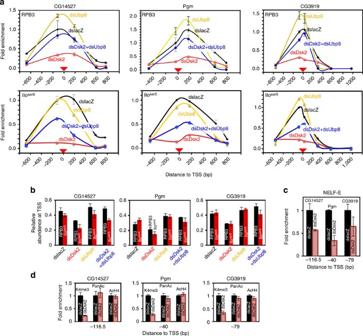Figure 7: dDsk2 regulates RNA pol II pausing at promoters of dHP1c complex target genes. (a) The levels of RPB3 (top) and the promoter-proximal Pol IIoser5form (bottom) across selected target genes are determined by ChIP–qPCR at the indicated positions with respect to TSS in control S2 cells treated with dsRNA against LacZ (black) and on depletion of dDsk2 (red), dUbp8/Nonstop (yellow) and both (blue). Results are presented as fold enrichment with respect to the control (dsLacZ) at the most proximal position to the TSS. The position of the TSS is indicated. Antibodies used were rabbit polyclonal αRPB3 and αIIoser5(N=3). (b) The relative abundance of RPB3 (black) and Pol IIoser5(red) at TSS with respect to their total abundance across the gene is determined for the indicated target genes in control S2 cells treated with dsRNA against LacZ and on depletion of dDsk2, dUbp8/Nonstop and both (N=3). (c) NELF-E levels at the indicated positions with respect to TSS of selected target genes are determined by ChIP–qPCR in control S2 cells treated with dsRNA against LacZ (black) and on depletion of dDsk2 (red). Results are presented as fold enrichment with respect to the control (dsLacZ). Antibodies used were rabbit αNELF-E antibodies (N=3). (d) H3K4me3 (left), acetylated H3 and H4 (PanAc; centre) and acetylated H4 (AcH4; right) levels at the indicated positions with respect to TSS of selected target genes are determined by ChIP–qPCR in control S2 cells treated with dsRNA against LacZ (black) and on depletion of dDsk2 (red). Results are presented as fold enrichment with respect to the control (dsLacZ). Antibodies used were rabbit polyclonal αH3K4me3, αPanAc and αAcH4 (N=3). Error bars correspond to s.d. Figure 7: dDsk2 regulates RNA pol II pausing at promoters of dHP1c complex target genes. ( a ) The levels of RPB3 (top) and the promoter-proximal Pol IIo ser5 form (bottom) across selected target genes are determined by ChIP–qPCR at the indicated positions with respect to TSS in control S2 cells treated with dsRNA against LacZ (black) and on depletion of dDsk2 (red), dUbp8/Nonstop (yellow) and both (blue). Results are presented as fold enrichment with respect to the control (dsLacZ) at the most proximal position to the TSS. The position of the TSS is indicated. Antibodies used were rabbit polyclonal αRPB3 and αIIo ser5 ( N =3). ( b ) The relative abundance of RPB3 (black) and Pol IIo ser5 (red) at TSS with respect to their total abundance across the gene is determined for the indicated target genes in control S2 cells treated with dsRNA against LacZ and on depletion of dDsk2, dUbp8/Nonstop and both ( N =3). ( c ) NELF-E levels at the indicated positions with respect to TSS of selected target genes are determined by ChIP–qPCR in control S2 cells treated with dsRNA against LacZ (black) and on depletion of dDsk2 (red). Results are presented as fold enrichment with respect to the control (dsLacZ). Antibodies used were rabbit αNELF-E antibodies ( N =3). ( d ) H3K4me3 (left), acetylated H3 and H4 (PanAc; centre) and acetylated H4 (AcH4; right) levels at the indicated positions with respect to TSS of selected target genes are determined by ChIP–qPCR in control S2 cells treated with dsRNA against LacZ (black) and on depletion of dDsk2 (red). Results are presented as fold enrichment with respect to the control (dsLacZ). Antibodies used were rabbit polyclonal αH3K4me3, αPanAc and αAcH4 ( N =3). Error bars correspond to s.d. Full size image Similar to dDsk2 depletion, depletion of dBre1 reduces H2Bub1 levels at TSS ( Figs 5f and 8a ) and downregulates expression of target genes ( P <0.01, Student’s t -test; Fig. 8b ). Thus, we also analysed its effect on RNA pol II pausing. As shown in Fig. 8c,d , dBre1 depletion does not significantly reduce RPB3 and Pol IIo ser5 levels at TSS, suggesting that pausing is not impaired. Co-depletion of dUbp8/Nonstop and dBre1 restores H2Bub1 levels ( Fig. 8a ) and maintains normal RPB3 and Pol IIo ser5 levels at TSS ( Fig. 8c,d ). However, it has little effect in the expression of target genes ( Fig. 8b ), which is in contrast to what is observed in dDsk2-depleted cells, where dUbp8/Nonstop co-depletion strongly rescues expression ( Fig. 6d ). 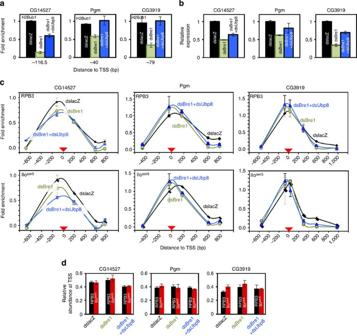Figure 8: dBre1 depletion does not affect RNA pol II occupancy at TSS. (a) H2Bub1 levels at the indicated positions with respect to TSS of selected target genes are determined by ChIP–qPCR in control S2 cells treated with dsRNA against LacZ (black) and on depletion of dBre1 (green) and co-depletion of dBre1 and dUbp8/Nonstop (blue). Results are presented as fold enrichment with respect to the control (dsLacZ). Antibodies used were mouse monoclonal αH2Bub1 (N=3). (b) mRNA levels of the indicated target genes are determined by RT–qPCR in S2 cells on depletion of dBre1 (green) and co-depletion of dBre1 and dUbp8/Nonstop (blue). mRNA levels were determined in relation to control cells treated with dsRNA against LacZ (black). Results were normalized with respect to Actin5C levels (N=3). (c) The levels of RPB3 (top) and the promoter-proximal Pol IIoser5form (bottom) across selected target genes are determined by ChIP–qPCR at the indicated positions with respect to TSS in control S2 cells treated with dsRNA against LacZ (black) and on depletion of dBre1 (green) and co-depletion of dBre1 and dUbp8/Nonstop (blue). Results are presented as fold enrichment with respect to the control (dsLacZ) at the most proximal position to the TSS. The position of the TSS is indicated. Antibodies used were rabbit polyclonal αRPB3 and αIIoser5(N=3). (d) The relative abundance of RPB3 (black) and Pol IIoser5(red) at TSS with respect to their total abundance across the gene is determined for the indicated target genes in control S2 cells treated with dsRNA against LacZ and on depletion of dBre1 and co-depletion of dBre1 and dUbp8/Nonstop (N=3). Error bars correspond to s.d. Figure 8: dBre1 depletion does not affect RNA pol II occupancy at TSS. ( a ) H2Bub1 levels at the indicated positions with respect to TSS of selected target genes are determined by ChIP–qPCR in control S2 cells treated with dsRNA against LacZ (black) and on depletion of dBre1 (green) and co-depletion of dBre1 and dUbp8/Nonstop (blue). Results are presented as fold enrichment with respect to the control (dsLacZ). Antibodies used were mouse monoclonal αH2Bub1 ( N =3). ( b ) mRNA levels of the indicated target genes are determined by RT–qPCR in S2 cells on depletion of dBre1 (green) and co-depletion of dBre1 and dUbp8/Nonstop (blue). mRNA levels were determined in relation to control cells treated with dsRNA against LacZ (black). Results were normalized with respect to Actin5C levels ( N =3). ( c ) The levels of RPB3 (top) and the promoter-proximal Pol IIo ser5 form (bottom) across selected target genes are determined by ChIP–qPCR at the indicated positions with respect to TSS in control S2 cells treated with dsRNA against LacZ (black) and on depletion of dBre1 (green) and co-depletion of dBre1 and dUbp8/Nonstop (blue). Results are presented as fold enrichment with respect to the control (dsLacZ) at the most proximal position to the TSS. The position of the TSS is indicated. Antibodies used were rabbit polyclonal αRPB3 and αIIo ser5 ( N =3). ( d ) The relative abundance of RPB3 (black) and Pol IIo ser5 (red) at TSS with respect to their total abundance across the gene is determined for the indicated target genes in control S2 cells treated with dsRNA against LacZ and on depletion of dBre1 and co-depletion of dBre1 and dUbp8/Nonstop ( N =3). Error bars correspond to s.d. Full size image Here we report that the extraproteasomal ubiquitin receptor dDsk2 interacts with the dHP1c complex, localizes at promoters and is required for transcription ( Figs 1 and 2 ). Binding sites of the dHP1c complex are marked by H2Bub1 and our results suggest that, through the UBA domain, dDsk2 binds H2Bub1 ( Fig. 5 ). However, reducing H2Bub1 levels affects binding of the complex only weakly ( Fig. 5f ), indicating that the interaction with H2Bub1 has only a minor contribution to recruitment. Actually, dDsk2 contains a single ubiquitin-binding site of low affinity ( K d ∼ 400 μM), which is in contrast to most ubiquitin receptors that contain several ubiquitin-binding sites that act synergistically to provide high-affinity binding [2] , [3] , [46] . Similarly, the interaction of dDsk2 with H2Bub1 is of low specificity since selective recognition of ubiquitylated substrates is largely based on the recognition of the linkage type, length and anchoring site of a polyubiquitin chain [2] , [3] , [46] , and, consequently, requires the presence of several ubiquitin-binding sites. In fact, the UBA domain of dDsk2 recognizes a monoubiquitylation in PTEN with a similar affinity as in H2B ( Fig. 5c ). On the other hand, binding of the dHP1c complex likely involves the recognition of specific DNA sequences since it depends on the zinc-finger proteins WOC and ROW [18] ( Supplementary Fig. 3a,b ). Noteworthy, dHP1c complex-binding sites are significantly enriched in a specific DNA sequence motif ( Supplementary Fig. 6 ). However, although the interaction with H2Bub1 is weak, binding of the complex unexpectedly depends on dDsk2 ( Supplementary Fig. 3c,d ). Besides, dHP1c is dispensable for WOC and ROW binding [18] , as well as for dDsk2 binding ( Supplementary Fig. 3a , bottom panel). These effects do not appear to be the consequence of changes in gene expression levels since dDsk2 mRNA levels do not significantly change on WOC, ROW or dHP1c depletion ( Supplementary Fig. 7 ). Furthermore, dDsk2 depletion upregulates ROW and weakly downregulates dHP1c mRNA levels ( Supplementary Fig. 7 ). Finally, it was reported that dHP1c interacts with RNA pol II [17] , [18] , [19] , suggesting that binding of the dHP1c complex might depend on RNA pol II. However, arguing against this possibility, we observed that binding of the complex at promoters is resistant to treatment with Actinomycin D ( Supplementary Fig. 8 ). Altogether, these results suggest that WOC, ROW and dDsk2 constitute the actual binding module of the complex, being fully interdependent for binding to chromatin and required for binding of dHP1c. In this regard, the slight reduction of ROW and dHP1c protein levels observed on dDsk2 depletion ( Fig. 4a,b ) is most likely due to their inability to bind chromatin, as described previously for dHP1c in ROW and WOC knockdowns [18] , as well as for other chromatin-associated proteins when their binding to chromatin is impaired [47] , [48] . Our results suggest that the main function of dDsk2 in the dHP1c complex is to prevent H2Bub1 deubiquitylation by dUbp8/Nonstop, as H2Bub1 levels are strongly reduced on dDsk2 depletion and recovered after dUbp8/Nonstop co-depletion ( Fig. 6c ). Protection against deubiquitylation has also been reported for Rad23 (refs 49 , 50 ) and appears to be a common feature of many ubiquitin receptors [10] , [11] . Simultaneous dDsk2 and dUbp8/Nonstop depletion also restores expression of target genes ( Fig. 6d ), whereas it has no effect on recruitment of the complex at promoters ( Fig. 6e ). Furthermore, overexpression of the ΔUBA–dDsk2 construct, which misses the UBA domain that mediates interaction with H2Bub1 in vitro ( Fig. 5b ), reduces H2Bub1 levels at promoters ( Fig. 6b ) and downregulates expression of target genes ( Fig. 5e ). Altogether, these results strongly suggest that the contribution of dDsk2 to transcription regulation is mainly based on this protective function. dHP1c complex target genes show features associated with strong RNA pol II pausing ( Fig. 3 ). Our results support a contribution of dDsk2 to pausing since its depletion reduces RNA pol II occupancy preferentially at TSS ( Fig. 7b ) and strongly decreases NELF-E levels ( Fig. 7c ). dDsk2 depletion downregulates expression ( Fig. 2f ) and, in good agreement, total RNA pol II occupancy across target genes is reduced ( Fig. 7a ). Interestingly, the majority of NELF target genes are also downregulated on NELF depletion in S2 cells [51] , and NELF potentiates gene expression in the Drosophila embryo [52] . Actually, ∼ 80% of dHP1c complex target genes that change expression in NELF knockdown conditions are downregulated. Furthermore, NELF-E depletion shows a similar reduction of total RNA pol II occupancy across target genes ( Supplementary Fig. 4 ). Altogether, these observations suggest that disrupting RNA pol II pausing does not generally increase productive transcription, but results in reduced total RNA pol II occupancy and decreased expression. It is possible that premature pause release interferes with RNA pol II activation into elongation, resulting in abortive transcription that, in turn, could affect RNA pol II recruitment and/or re-initiation. Notice, however, that dDsk2 depletion does not affect the extent of histone acetylation detected at target promoters ( Fig. 7d ), suggesting that they retain the transcriptional active chromatin state. Notably, co-depletion of dUbp8/Nonstop, which rescues H2Bub1 ( Fig. 6c ), also rescues the pausing defect caused by dDsk2 depletion ( Fig. 7a,b ) and expression levels are restored ( Fig. 6d ), suggesting that dynamic regulation of H2Bub1 levels at promoters of dHP1c target genes plays a role in RNA pol II pausing. In this regard, work performed in yeast suggested that transcriptional activation involves sequential cycles of H2B ubiquitylation and deubiquitylation [32] and that Ubp8 promotes Ctk1-dependent phosphorylation of Ser2 in the CTD [33] , a modification that is required for activation into the elongating Pol IIo ser2 form. Nevertheless, H2Bub1 deubiquitylation at TSS does not appear to be sufficient by itself to induce pause release since dBre1 depletion, which also reduces H2Bub1 at TSS ( Figs 5f and 8a ), has no significant effect in pausing ( Fig. 8c,d ). In this regard, it must be noted that dBre1 travels with the elongating RNA pol II along coding regions to induce H2Bub1, which stimulates Facilitates-Chromatin-Transcription (FACT) activity and, thus, facilitates elongation [29] , [30] , [31] , [53] . On the other hand, dUbp8/Nonstop activity is mainly restricted to promoters since its depletion in dBre1-deficient cells has little effect in H2Bub1 levels at coding regions ( Supplementary Fig. 9 ). On the contrary, dUbp8/Nonstop depletion in dDsk2-deficient cells strongly rescues H2Bub1 levels at coding regions ( Supplementary Fig. 9 ). Interestingly, whereas dUbp8/Nonstop depletion restores expression of target genes in dDsk2-depleted cells ( Fig. 6d ), it has only a slight effect in dBre1-deficient cells ( Fig. 8b ). Altogether, these results suggest that dBre1 depletion impairs elongation and, thus, might prevent the release of paused RNA pol II by disturbing its actual engagement into elongation. Further work is required to better understand the mechanisms that regulate RNA pol II pausing, the actual contribution of dDsk2 and whether it involves H2Bub1 and/or additional factors also targeted by ubiquitylation. The dHP1c complex appears to have a particularly important contribution to nervous system development and function since target genes are enriched in related functions ( Fig. 3a ) and knockdown conditions preferentially affect gene expression in the nervous system [18] . Actually, WOC and ROW are highly expressed in the nervous system during embryo and larval development, and mutant larvae show brain defects [54] , [55] . Furthermore, in humans, the WOC homologue DXS6673E/ZNF261 has been implicated in X-linked mental retardation [56] . Interestingly, mutations in the human Dsk2 homologues (Ubqln-1/2) have been associated with Alzheimer’s disease as well as other neurodegenerative diseases [57] . Noteworthy, Ubqln-1/2 are detected in both the nucleus and the cytoplasm, and the development and progression of neurofibrillary tangles in Alzheimer’s disease brains associate with an altered nuclear Ubqln-1 content [58] . Whether the role of dDsk2 in transcription regulation is conserved in humans and contributes to disease remains to be determined. In summary, our results indicate that the ubiquitin receptor dDsk2 plays a nonproteolytic function in the regulation of H2Bub1 and RNA pol II pausing at promoters of dHP1c complex target genes. Ubiquitin receptors have been previously reported to play nonproteolytic functions in DNA repair and transcription elongation [6] , [7] , [8] , [9] . Furthermore, in response to DNA damage, human Rad23B was found to interact with ubiquitylated p53, localize at chromatin and accumulate at the p21 promoter [59] . In addition, in mouse embryonic stem cells, several components of the NER complex, including Rad23B, have been shown to act as an Oct4/Sox2 co-activator complex that associates with chromatin and is required for stem cell maintenance [60] . Recruitment of NER factors to active promoters has also been reported in HeLa cells in the absence of DNA damage [61] . However, in these cases, the precise function of the ubiquitin receptor has not been elucidated. In this regard, our results expand the catalogue of nonproteolytic functions of ubiquitin receptors to the epigenetic regulation of chromatin modifications and transcription initiation. It must also be noted that ubiquitylation participates in the regulation of multiple genomic functions and that the number of proteins containing ubiquitin-binding domains is large, ∼ 100 in humans. Therefore, a role of ubiquitin-binding proteins as epigenetic regulators of chromatin emerges as a distinct possibility. Drosophila stocks and genetic procedures hp1c RNAi , row RNAi and woc RNAi lines are described in ref. 18 . dsk2 RNAi was obtained from the Vienna Drosophila Resource Center (VDRC) and correspond to line 47448. act5C -GAL4, ptc -GAL4 and lio -GAL4 were obtained from the Bloomington Stock Center. For RNAi depletion, crosses were set up at 25 °C and moved to 29 °C 3 days before dissection. Efficiency of depletion by hp1c RNAi , row RNAi and woc RNAi is reported in ref. 18 . Efficiency of depletion by dsk2 RNAi was determined by immunostaining with αdDsk2 antibodies in polytene chromosomes ( Supplementary Fig. 10 ) and wing imaginal discs ( Fig. 4b ). Antibodies Polyclonal rabbit αHP1c (ChIP/IP: 5 μl) and αHP1b (ChIP/IP: 5 μl) were custom made by ABGENT against peptides aa143–157 and aa219–233, respectively. Polyclonal rat αWOC (IF: 1/500) and rabbit αROW (WB: 1/10,000, ChIP/IP: 1 μl) antibodies were raised against recombinant proteins aa230–626 and aa588–956, respectively. Other antibodies used are described in the indicated references: rat αHP1c (WB: 1/10,000, IF: 1/500, ChIP/IP: 1 μl), αHP1b (WB: 1/10,000, ChIP/IP: 1 μl) and αROW (WB: 1/10,000, IF: 1/400, ChIP/IP: 1 μl) [18] , rabbit αWOC (WB: 1/10,000, ChIP/IP: 1 μl) [62] , rabbit and rat αDDP1 (ChIP/IP: 1 μl) [63] , rabbit αdDsk2 (WB: 1/12,000, IF: 1/1,000, ChIP/IP: 1 μl) [16] , mouse αp54 (WB: 1/50) [64] , rabbit αNELF-E (WB: 1/500, ChIP/IP: 3 μl) [65] and rabbit αRPB3 (WB: 1/1,500, ChIP: 15 μl) [26] . Commercially available antibodies used were as follows: rabbit αH3K4me3 (Abcam, ab8580, ChIP: 1 μl), rabbit αIIoser5 (Abcam, ab5131, ChIP: 3 μl), rabbit αBre1 (NOVUS, 40280002, WB: 1/1,000, ChIP: 2 μl) and αRad6 (SANTA CRUZ, sc-30078, WB: 1/500, ChIP: 2 μl), mouse αGST (glutathione S-transferase; Novagen, 71097-3, WB: 1/10,000), mouse αGFP (Roche, 1814460, IF: 1/50), mouse αH2Bub1 (Millipore, 05–1312, WB: 1/4,000, ChIP/IP: 1 μl), mouse αTubulin (Millipore, MAB3408, WB: 1/2,000), rabbit αActin (Sigma, A2066, WB: 1/10,000), mouse αV5 (Invitrogen, 460705, WB: 1/5,000), mouse αUbiquitin (SANTA CRUZ, sc-8017, WB: 1/500), rabbit αPanAc (Abcam, Ab193–100, ChIP: 1 μl) and rabbit αH4Ac (Millipore, no. 06–866, ChIP: 1 μl). Dilutions used in immunostaining (IF), ChIP, IP and WB experiments are indicated. Constructs Full-length Row -coding sequence was cloned into pMK33-C-TAP . Full-length Woc -coding sequence was cloned into pMK33-NTAP . dDsk2 full-length and deletion constructs were generated using the pAc5.1/V5-HisA (Invitrogen) and the pGEX-2TK (Amersham) vectors. dDsk2–ΔUbL is lacking aa1–80, dDsk2–ΔUBA is lacking aa496–547 and dDsk2–UBA corresponds to aa469–547. Complex purification and characterization Stable S2 cell lines were generated using the plasmids pMK33-ROW-TAP and pMK33-TAP-WOC . TAP-tagged expression was induced by overnight treatment with 0.07 mM CuSO 4 . Crude nuclear extracts were prepared according to conventional methods and precleared by incubation with BSA Dynabeads (Invitrogen) for 1 h at 4 °C. Then, the precleared extracts were incubated with IgG Dynabeads for 4 h at 4 °C in Buffer B (20 mM HEPES pH 7.9, 20% Glycerol, 0.3 M NaCl, 3 mM MgCl 2 , 1 mM EGTA and 1 mM dithiothreitol (DTT), Protease Inhibitor Cocktail). After incubation, the beads were extensively washed with Wash Buffer (20 mM HEPES pH 7.9, 20% Glycerol, 0.3 M NaCl, 0.1% NP-40, 0.5 mM EGTA and 0.5 mM DTT, Protease Inhibitor Cocktail). Elution was performed with 50 mM Glycin-HCl pH3. Aliquots were checked with SDS–PAGE and silver staining. The remaining eluate was run into a stacking gel, from where a single band was cut and interacting proteins were identify using LC/MS at the Proteomics Unit of the ‘Institut de Recerca de la Vall d’Hebron’ Barcelona. Co-IP experiments Co-IPs were performed using extracts from S2 cells or transiently transfected S2 cells with dDsk2-V5 expression constructs. Cells were lysed in IP buffer (50 mM Tris-HCl pH 8, 250 mM NaCl, 5 mM EDTA, 0.5% NP-40 and Protease Inhibitor cocktail). Extracts were incubated with antibodies in IP buffer overnight at 4 °C. Then, Protein A sepharose (GE Healthcare) or Protein G agarose (Santa Cruz Biotechnology) was added and further incubated at 4 °C for 2 h. After several washes with IP buffer, the beads were eluted in SDS-loading buffer and the results were analysed using WB analysis. Glycerol gradient sedimentation Total soluble extracts were prepared from S2 cells in 225 mM NaCl, 50 mM Tris-HCl pH 8, 5 mM EDTA, 0.5% NP-40, 0.1 mM phenylmethylsulphonyl fluoride (PMSF) and Protein Inhibitor Cocktail, and 250 μl of extract were loaded on a 12-ml 10–30% glycerol gradient in 10 mM Tris-HCl pH 8, 100 mM KCl, 12.5 μM EDTA. Centrifugation was carried out in an SW40.1ti rotor at 35,000 r.p.m. (RCFmax=217,874 × g ) for 20 h at 4 °C. Fractions of 350 μl were collected from the top of the gradient and analysed using WB analysis. Pull-down assays For peptide pulldowns, 2 μg of the corresponding GST construct and 0.25 nmol of the corresponding biotinylated peptide were incubated overnight at 4 °C with streptavidin sepharose in peptide-binding buffer (50 mM Tris-HCl pH 8, 100 mM NaCl, 0.1% NP-40, 1 mM DTT and Protease Inhibitor Cocktail) in a total volume of 500 μl. Then, the beads were washed three times with 1 ml peptide-binding buffer and eluted in SDS-loading buffer. The results were analysed with WB analysis using mouse αGST. Custom-made N-terminally biotinylated Drosophila H2B peptides corresponding to aa104–124 either ubiquitylated (H2BubK118) or unmodified at K118 (H2BK118) were purchased from UbiQ. To determine the specificity of the binding of the UBA domain of dDsk2 to H2Bub1, we performed GST pull-down assays. In this case, glutathione sepharose 4B beads were incubated with the GST–UBA construct in the presence of either the H2BubK118 peptide or a PTENubK13 peptide (aa5–21) ubiquitylated at K13 (LifeSensors, UP100). Binding was analysed with WB analysis using mouse αUbiquitin (Santa Cruz). Overexpression experiments For overexpression experiments, 3 million cells were seeded in 5 ml dishes and cultured overnight. Then, each dish was transfected using the CaCl 2 precipitation method with 24 μg of plasmid DNA: empty pAc5.1 (control), pAc5.1-Dsk2 full-length (Dsk2) or pAc5.1-Dsk2 (1–495) (ΔUBA–Dsk2). Cells were collected 48 h after transfection. Cellular fractionation S2 cells were collected 2 days after transient transfection of the indicated constructs and spun down for 5 min at 1,000 g . The cell pellet was washed two times with PBS. The pellet was then resuspended in Buffer A (10 mM HEPES pH 7.9, 10 mM KCl, 1.5 mM MgCl 2 , 0.34 M Sucrose, 10% Glycerol, 1 mM DTT and Protease Inhibitor cocktail). Triton X-100 was added to final 0.1% and the sample was gently mixed and incubated on ice for 8 min. Then, centrifugation was carried out for 5 min at 1,300 g resulting in pellet P1 (nuclei) and supernatant S1. To obtain the cytosolic fraction S1 was clarified by centrifugation at 16,000 g for 10 min. The pellet P1 was washed in Buffer A and then lysed for 30 min in Buffer B (10 mM HEPES pH 7.9, 3 mM EDTA, 0.2 mM EGTA, 1 mM DTT and Protease Inhibitor Cocktail). Then, centrifugation was carried out at 1,700 g for 5 min resulting in supernatant S3 (soluble nuclear fraction) and in pellet P3. After washing P3 with Buffer B, pellet P4 (chromatin) was obtained. The total extracts were prepared in parallel by lysing pellets of S2 directly in SDS-loading buffer. Equivalent amounts of total extracts and cellular fractions were analysed using WB analysis. Immunostaining experiments Immunostaining experiments were performed in polytene chromosomes and imaginal discs of third instar larvae according to ref. 18 . For visualization, slides were mounted in Mowiol (Calbiochem-Novabiochem) containing 0.2 ng ml −1 DAPI (Sigma) and visualized in a Nikon Eclipse E-800 inverted microscope. RNAi knockdown experiments in S2 cells dsRNA was prepared using the MEGAscript T7 kit (Ambion). For knockdown in S2 cells, cells were diluted to 10 6 ml −1 and incubated for 2 days with 4 μg dsRNA per 10 6 cells. Then, they were diluted again to 10 6 ml −1 and incubated for 3 more days after addition of another 4 μg dsRNA per 10 6 cells. Then, cells were collected and used for consecutive experiments. An aliquot was taken to check the knockdown efficiency using WB analysis ( Supplementary Fig. 11 ). Notice that rabbit polyclonal αWOC does not give rise to any specific signal. Therefore, in this case, the extent of depletion was determined from the destabilization of dHP1c observed when its binding to chromatin is impaired in the absence of WOC or ROW [18] . Primers used for dsRNA production are described in Supplementary Table 1 . Expression profiling and RT–qPCR experiments For expression profiling analyses, total RNAs were prepared from control S2 cells and on RNAi-mediated depletion of ROW, converted to cDNA, hybridized to Drosophila Genome 2.0 GeneChip (Affymetrix) and analysed essentially as described in ref. 66 . Microarray data were deposited in the NCBI Gene Expression Omnibus repository (GSE49103). To assess differential expression, we used the limma-moderated t -test statistics to compute posterior probabilities of differential expression, following the empirical Bayes semiparametric procedure described in ref. 67 and setting the false discovery rate at 0.05. NELF knockdown microarray data were downloaded from NCBI GEO (GSE6141) [51] . For expression analysis of selected target genes by RT–qPCR, RNA was prepared from S2 cells using a combination of Trizol (Ambion) and RNeasy mini kit (Qiagen). RNA was retro-transcribed using the Transcriptor First Strand cDNA Synthesis Kit (Roche) with oligo (dT) 18 primers. Real-time PCR was performed using the standard curve method. Normalization was carried out against the control gene α Tubulin and then fold change of RNA levels in mutants were represented relative to RNA levels in dslacZ-treated S2 cells. Primers used in these experiments are described in Supplementary Table 1 . WB analyses WB analyses were performed according to conventional methods. Full scans of the WB presented in Figures and Supplementary Figures are shown in Supplementary Fig. 12 . ChIP experiments For preparing chromatin for ChIP, S2 cells were crosslinked for 10 min by adding 1.8% formaldehyde directly to the media and incubating on the shaker at room temperature. Glycin (125 mM) was added to stop the reaction. Cells were washed once each with PBS, Wash Buffer A (10 mM HEPES pH 7.9, 10 mM EDTA, 0.5 mM EGTA and 0.25% Triton X-100) and Wash Buffer B (10 mM HEPES pH 7.9, 100 mM NaCl, 1 mM EDTA, 0.5 mM EGTA and 0.01% Triton X-100). The pellet was then resuspended in TE and 1% SDS was added, followed by centrifugation at 1,500 g . The supernatant was carefully removed and two washes with TE were performed. Then TE buffer, 0.1% SDS and 1 mM PMSF were added. Sonication was performed using the 15-ml tube holder of a Bioruptor sonicator. A total of 25 sonication cycles of 30 s ON/30 s OFF were performed at high intensity. After sonication, 1% Triton X-100, 0.1% deoxycholate and 140 mM NaCl were added. Samples were cleared using centrifugation and aliquots were stored at −80 °C. Before performing the ChIP, chromatin samples were precleared for 1 h with Protein A sepharose. Antibody was added to the precleared chromatin and rotated overnight at 4 °C. Protein A sepharose was added and incubation was continued for 3 h. Five washes with RIPA buffer (140 mM NaCl, 10 mM Tris-HCl pH 8, 1 mM EDTA, 1% Triton X-100, 0.1% SDS and 0.1% Deoxycholate), one wash with LiCl ChIP buffer (250 mM LiCl, 10 mM Tris-HCl pH 8, 1 mM EDTA, 0.5% NP-40 and 0.5% Deoxycholate) and two washes with TE buffer were performed. After RNAse treatment, elution was performed in 0.1 M NaHCO 3 , 1% SDS and by extensive vortexing. Eluates were de-crosslinked overnight at 65 °C. Then, samples were treated with Proteinase K and a Phenol–Chloroform DNA extraction followed by EtOH precipitation was performed. For ChIP–qPCR, triplicated samples were analysed using the standard curve method. Normalization was performed with respect to the corresponding control sample. Primers used in these experiments are described in Supplementary Table 1 . Relative abundance at TSS was determined by calculating the proportion of Rpb3 (or Pol IIo ser5 ) detected at the peak position, as compared with the total amount of Rpb3 (or Pol IIo ser5 ) detected at all the analized positions along the gene. For ChIP-seq, 10 ng of DNA, quantified with the Qubit dsDNA HS Assay Kit (Invitrogen) was used for library preparation. End-repair, adenylation, ligation of adapters and PCR enrichment for 18 cycles were performed using TruSeqRNA Sample Prep Kit (Illumina) according to the manufacturer’s recommendations. Purified libraries were quantified with the Qubit dsDNA HS Assay Kit (Invitrogen) and size distribution was evaluated using the Bioanalyzer DNA 1000 assay (Agilent). Single-end sequencing of 50 nucleotides was performed on the Genome Analyzer IIx. For treatment with Actinomycin D, 15 × 10 6 cells were seeded in 15 ml of medium, grown for 48 h and then treated for 30 min with 1 μg ml −1 Actinomycin D (Sigma A1410) or dimethylsulphoxide, as control, and then processed for ChIP-qPCR as described above. Bioinformatics and biostatistics analyses Except where otherwise indicated, all analyses were performed with the Bioconductor software. For analysis of ChIP-seq data, Solexa/Illumina sequencing data for WOC, ROW, dHP1c and dDsk2 were pre-processed with the standard Illumina pipeline version 1.5.1. Sequence alignment to the Drosophila melanogaster genome (UCSC dm3 version) and binding site determination were performed essentially as described in ref. 66 setting the coverage difference between IP and the corresponding input sample to 30 reads for WOC and ROW, and 20 reads for dHP1c and dDsk2. ChIP-Seq profiles and binding sites were deposited in the NCBI Gene Expression Omnibus repository (GSE49102). Binding sites were assigned to overlapping and closest genes using the UCSC refflat gene annotations ( http://hgdownload.cse.ucsc.edu/goldenPath/dm3/database/refFlat.txt.gz ; April 2013) considering the longest possible transcript for each gene and using the annotatePeakInBatch from the ChIPpeakAnno Bioconductor package for annotation. Distance to overlapping and closest genes was measured from the midpoint of the peak to the gene TSS. To determine the distribution of ChIP-seq reads around the TSS, we plotted the average read coverage using the function plotMeanCoverage in the Bioconductor package htSeqTools. Peak density around loci of interest was plotted using the PeakLocation function from the htSeqTools package. Gene ontology (GO) and KEGG enrichment pathway analyses were performed as described in ref. 66 and statistical significance assessed with Fisher’s exact test, with Benjamini–Yekutieli multiple testing adjustment. When dHP1c abundance at WOC/ROW/dHP1c target genes was compared with abundance at WOC/ROW target and non-target genes, we computed the reads per kilobase per million (RPKM) as 10 6 R /( ML ), where R is the number of reads mapped to a given gene, M is the total number of reads and L is the distance between TSS and TES in kb. ChIP-on-chip-binding site data for dHP1b, dHP1c and H2Bub1 were obtained from modENCODE (IDs 941, 3291 and 290) and ChIP-seq-binding site data for Pol IIo Ser5 from NCBI GEO (GSE19325) [68] . ChIP-on-chip data for NELF-E were downloaded from ArrayExpress (E-MEXP-1547) [69] and binding sites were determined with the rMAT package. First, arrays were normalized using the NormalizeProbes function with the PairBinned method. Then, probe intensity scores were computed with the computeMATScore function, setting the dMax option to 150. Finally, binding sites were detected as enriched regions with the callEnrichedRegions function, using the following options: dMax=150, dMerge=150, nProbesMin=8, and setting the false discovery rate threshold at 0.01. Binding sites were annotated to the D. melanogaster reference genome as described above for ChIP-seq peaks. Peak density plots were produced using the PeakLocation function from the htSeqTools package. Total RNA pol II (RPB1) ChIP-Seq data (reads and binding sites) were downloaded from NCBI GEO (GSE32120) [70] . Binding sites were annotated as described above. Standardized peak density plots were determined using the StdPeakLocation function in the htSeqTools package. The PI was computed for all genes longer than 500 bp as the ratio between RPKM detected within ±250 bp around the TSS and in the last 500 bp of the gene [24] . Statistical significance for PI difference was assessed using the Kruskal–Wallis test. Genome-wide data for KMnO 4 reactivity were downloaded from NCBI GEO (GSE46620) [27] . First, reactive sites were defined as those with a Thymine-reactivity score ( T -score) above the third quartile and annotated for overlapping genes as described before. Per-gene T -score was computed as the sum of T -score values across the whole gene and normalized by gene length. Genes were then classified according to the resulting score as low (min to first quartile), medium (first to third quartile) or high (third quartile to max), to assess the proportion of identified targets within each KMnO 4 reactivity score gene set. Benjamini–Yekutieli adjusted P values for the observed proportion differences were computed with the Fisher’s exact test. shortRNA-Seq data were downloaded from NCBI GEO (GSE18643) [26] . shortRNA sites were defined as those with a score above the third quartile and annotated for overlapping genes as described above. Accession codes: ChIP-seq and Microarray data generated in these experiments are deposited in GEO under the accession code GSE49104 . How to cite this article: Kessler, R. et al. dDsk2 regulates H2Bub1 and RNA polymerase II pausing at dHP1c complex target genes. Nat. Commun. 6:7049 doi: 10.1038/ncomms8049 (2015).